The molecular landscape of colorectal cancer cell lines unveils clinically actionable kinase targets The development of molecularly targeted anticancer agents relies on large panels of tumour-specific preclinical models closely recapitulating the molecular heterogeneity observed in patients. Here we describe the mutational and gene expression analyses of 151 colorectal cancer (CRC) cell lines. We find that the whole spectrum of CRC molecular and transcriptional subtypes, previously defined in patients, is represented in this cell line compendium. Transcriptional outlier analysis identifies RAS/BRAF wild-type cells, resistant to EGFR blockade, functionally and pharmacologically addicted to kinase genes including ALK, FGFR2, NTRK1/2 and RET. The same genes are present as expression outliers in CRC patient samples. Genomic rearrangements (translocations) involving the ALK and NTRK1 genes are associated with the overexpression of the corresponding proteins in CRC specimens. The approach described here can be used to pinpoint CRCs with exquisite dependencies to individual kinases for which clinically approved drugs are already available. Knowledge of tumour biology and the development of new anticancer agents depend on robust preclinical model systems that reflect the genomic heterogeneity of human cancers and for which detailed genetic and pharmacologic annotations are available. Cell lines represent a mainstay to functionalize molecular data as they allow experimental manipulation, global and detailed mechanistic studies and high-throughput applications [1] , [2] , [3] , [4] . Virtually all commonly used cancer cells were continuously grown in vitro for years, and decades have often passed since they were originally derived from patients. The in vitro culture conditions used to propagate cancer cells are far from the histological landscape in which they originated. These considerations are often cited to question the relevance of cell lines as cancer models. We further observe that, for a given cancer type, only few cell lines (<10) are employed in most preclinical studies. The evidence that cancer patients have heterogeneous genetic features implies that a large number of lineage-specific cell lines is needed to capture the diversity observed in the clinic. Furthermore, cells commonly used to model a tumour type may not represent the patients that they intend to recapitulate. For instance, colorectal cancer (CRC) cell lines ordinarily used in preclinical studies often display microsatellite instability (MSI). MSI colorectal tumours are found in 10–15% patients [5] , but they show an indolent clinical behaviour and are less prevalent in more advanced stages of the disease, accounting for <5% in the metastatic setting [6] , [7] . Consequently, MSI cell lines do not properly recapitulate the clinical setting in which targeted agents are most commonly administered to CRC patients. In addition to the ‘genetic’ driven subtypes, tumour lineages can be subdivided based on their transcriptional profiles. Transcriptional profiling has been recently used to identify distinct CRC subtypes [8] , [9] , [10] , [11] , [12] . The subtypes are associated with biological and clinical features such as cell of origin, MSI, prognosis and response to treatments. Whether the transcriptional subtypes are maintained in CRC cell models and how this knowledge can be used to discover novel pharmacogenetic relationships has not been explored. To address these challenges, we assembled and annotated a comprehensive collection of 151 human CRC cells. We find that the molecular heterogeneity (oncogenic mutations and transcriptional subtypes), previously defined in CRC patients, is maintained in CRC cells. Individual lines can be stratified as responders or non-responders to epidermal growth factor receptor (EGFR) blockade based on clinically validated biomarkers. Transcriptional outlier analysis identifies CRC cells, resistant to EGFR blockade, pharmacologically addicted to kinase genes including ALK , FGFR2 , NTRK1/2 and RET . Genetic and transcriptional profiling of CRC cells A collection of 152 CRC cell lines was initially genotyped at 10 different microsatellite loci (short tandem repeat (STR) profile) to unequivocally define their genetic identities ( Supplementary Data 1 ). This analysis revealed that a few cell lines, previously thought to be unrelated, were derived from the same patient ( Supplementary Data 1 ). Global mRNA expression profiling was carried out on the entire cell bank and TiGER (tissue-specific gene expression database) [13] was exploited to perform a ‘tissue of origin’ analysis ( Supplementary Fig. 1a ). The analysis revealed a probable non-intestinal origin for one line, COLO741, found to express skin-specific genes, including Tyrosinase ( Supplementary Fig. 1b,c ). This, together with the lack of expression of the neuroendocrine markers CHGA, SYP, ENO2, ACPP and NCAM1, suggested that these cells are not derived from a CRC nor from a neuroendocrine tumour, but rather from a melanoma. For this reason, COLO741 cells were withdrawn from further analyses. HuTu80 cells displayed a small intestine-like signature ( Supplementary Fig. 1d ) and were included in subsequent analyses due to their intestinal origin. Gene expression-based hierarchical clustering revealed that cell lines with identical genetic background consistently clustered together ( Fig. 1 ), indicating that the genotype maintained strong control over the transcriptome. The only exception was the COGA5/COGA5L pair; these lines were derived respectively from the primary tumour and a lymph node metastasis of the same patient [14] . 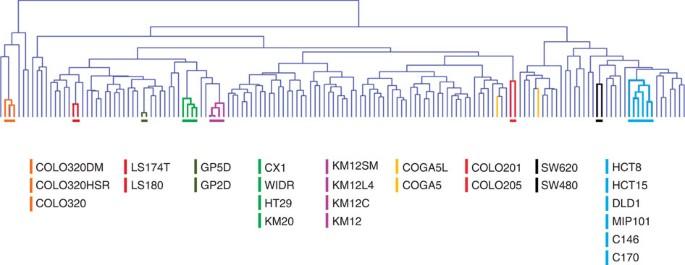Figure 1: Expression clustering of 151 CRC cell lines. Unsupervised hierarchical clustering of 151 CRC cell lines based on their global expression profile. Cell lines derived from the same individual (same STR) are highlighted by the same colour. Names of the cell lines with identical STR are reported below the dendrogram in the order by which they occur in the cluster, from left to right. Figure 1: Expression clustering of 151 CRC cell lines. Unsupervised hierarchical clustering of 151 CRC cell lines based on their global expression profile. Cell lines derived from the same individual (same STR) are highlighted by the same colour. Names of the cell lines with identical STR are reported below the dendrogram in the order by which they occur in the cluster, from left to right. Full size image The 151 CRC cell line collection was then assessed for the occurrence of MSI. MSI was detected in 63/151 cases (42%; Supplementary Data 1 ). It has been previously noted that a higher than expected fraction of CRC cell lines are MSI, conceivably because MSI tumours can be more easily propagated in vitro [15] . We also observed that the rare hypermutator/MSI-negative subgroup, identified in about 2% of CRC cases, is represented by three lines, HT115, HCC2998 and HT55 (ref. 16 ). The mutational status of KRAS , NRAS , BRAF and PIK3CA was next assessed as these genes are implicated in the response of CRC to EGFR-targeted therapies and are often ascertained in the clinic ( Supplementary Data 1 ). KRAS , NRAS and BRAF mutations were mutually exclusive and were present in 47, 0.7 and 18% of the lines, respectively. PIK3CA mutations and absence of PTEN expression were detected in 18 and 14% of the cells, respectively, and occurred together with KRAS and BRAF at rates comparable to those previously reported [17] , [18] , [19] ( Supplementary Data 1 ). Overall, the complexity reached in this compendium effectively reflects the genetic heterogeneity recognized in sporadic CRCs. Sensitivity to cetuximab is an intrinsic trait of CRC cells The anti-EGFR monoclonal antibodies cetuximab or panitumumab are approved to treat metastatic CRC but achieve <10% objective response rates in unselected CRC patients when given in monotherapy [20] . Clinical benefit to EGFR blockade is confined to 25% of cases carrying tumours wild-type for KRAS , NRAS and BRAF [21] . To assess whether CRC lines recapitulated the above pharmacogenetic relationships, we determined sensitivity to cetuximab in the entire cell collection over a wide range of drug concentrations ( Fig. 2 , Supplementary Fig. 2 and Supplementary Data 1 ). Ten RAS/BRAF wild-type cell lines (7% of the total or 20% of RAS/BRAF wild-type cells) were highly susceptible to cetuximab inhibition ( Fig. 2 , Supplementary Fig. 2a ). Pharmacological parameters such as the area under the curve (AUC) or the percentage of cell growth inhibition at a clinically relevant drug concentration of 10 μg ml −1 (ref. 22 ) closely paralleled the response rates observed in patients [20] , [21] ( Supplementary Fig. 3a ). Cells classified as sensitive died on anti-EGFR treatment ( Supplementary Fig. 3b–d ), while partially sensitive cells were mainly growth impaired ( Supplementary Fig. 3e ). As observed in the clinical setting, KRAS , BRAF or NRAS mutations conferred complete resistance to EGFR blockade in CRC cells (Fisher exact text P value <0.001; Fig. 2 ). 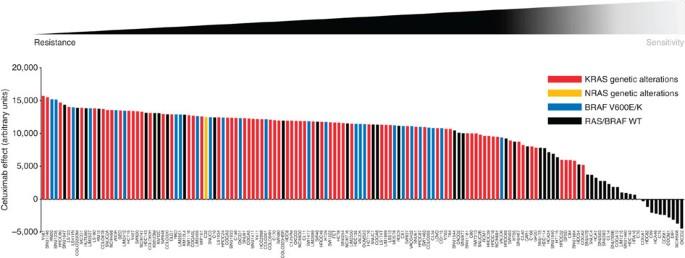Figure 2: Cetuximab screening on CRC cell lines. The indicated cell lines were treated with increasing concentrations of cetuximab for 4 days and the cell viability was assessed by measuring ATP content. Bars represent an arbitrary index of cetuximab effect on each cell line as detailed in the methods. Cell lines sensitive to cetuximab are shown with a negative index. Red bars representKRASaltered lines; yellow bars indicateNRAS-mutated cells; blue bars indicate genetic alterations affecting codon V600 ofBRAF; black bars indicateRAS/BRAFwild-type cells. NCIH630 cells areKRASamplified46. Figure 2: Cetuximab screening on CRC cell lines. The indicated cell lines were treated with increasing concentrations of cetuximab for 4 days and the cell viability was assessed by measuring ATP content. Bars represent an arbitrary index of cetuximab effect on each cell line as detailed in the methods. Cell lines sensitive to cetuximab are shown with a negative index. Red bars represent KRAS altered lines; yellow bars indicate NRAS -mutated cells; blue bars indicate genetic alterations affecting codon V600 of BRAF ; black bars indicate RAS/BRAF wild-type cells. NCIH630 cells are KRAS amplified [46] . Full size image CRC molecular subtypes are maintained in cell lines Colorectal tumours can be classified in up to six unique subtypes with diverse clinical features according to the genes they express [8] , [9] , [10] , [11] , [12] . To what extent the transcriptional subtypes are cell intrinsic or depend on the microenvironment is unclear. Expression profiles were therefore used to assign each cell line to a molecular subtype [8] , [9] , [10] , [11] , [12] by the Nearest Template Prediction (NTP) algorithm, which also estimates the classification false discovery rate (FDR) [23] . Each of the five classifiers was able to assign (FDR<0.2) the large majority of the cell lines to a subtype. Classifications of cell lines according to the five systems, together with the respective FDRs, are reported in Supplementary Data 2 . Significant overlaps were detected among distinct classifiers. We found that the CRC-assigner (CRCA) classification system established by Sadanandam et al. [12] shared the highest overlap with all other classifiers ( Supplementary Fig. 4a ). It was therefore considered as a reference for reconciling the five classifiers into a unified consensus ( Supplementary Fig. 4b ). Molecular and pharmacological associations, which previously emerged in CRC samples using the CRCA-based classification, were recapitulated in the cell collection ( Fig. 3 ). MSI cells were significantly enriched in inflammatory and goblet subtypes ( P values: 0.0334 for inflammatory, 0.008 for goblet) and less prevalent in the Transit Amplifying (TA) and Stem groups, which were instead mainly composed of microsatellite stable (MSS) cell lines ( P value<0.0005). BRAF -mutated cell lines clustered in the inflammatory subtype ( P value=0.0005), while RAS mutations were equally distributed among subgroups. Notably, six out of nine RAS/BRAF wild-type cetuximab-sensitive cells belonged to the TA subtype ( P =0.038). Such enrichment is in line with data on CRC specimens [12] ( Fig. 3 ). 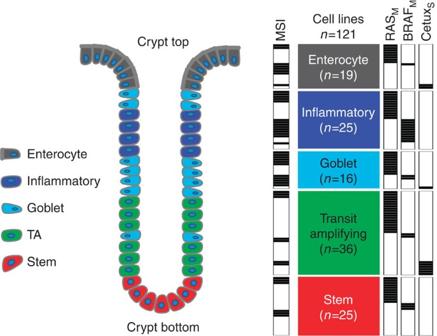Figure 3: CRC transcriptional subtypes are maintained in cell lines. CRC cell lines are classified according to the ‘CRC-assigner’ intrinsic transcriptional subtypes and the colon crypt location previously described12. MSI status,RAS/BRAFmutations and cetuximab sensitivity are indicated. The figure includes only CRC cell lines that were assigned to a subtype with FDR<0.2. Among cell lines sharing the same STR profile, we selected the original cell line in case of groups of cells including also derived clones, and in the absence of such information, the one classified with the highest confidence by the NTP algorithm. Cetux, cetuximab; BRAFM,BRAF-mutated cells; RASM,RAS-mutated cells. Figure 3: CRC transcriptional subtypes are maintained in cell lines. CRC cell lines are classified according to the ‘CRC-assigner’ intrinsic transcriptional subtypes and the colon crypt location previously described [12] . MSI status, RAS/BRAF mutations and cetuximab sensitivity are indicated. The figure includes only CRC cell lines that were assigned to a subtype with FDR<0.2. Among cell lines sharing the same STR profile, we selected the original cell line in case of groups of cells including also derived clones, and in the absence of such information, the one classified with the highest confidence by the NTP algorithm. Cetux, cetuximab; BRAF M , BRAF -mutated cells; RAS M , RAS -mutated cells. Full size image Outlier tyrosine kinases overexpressed in CRC cells To unveil actionable targets likely to be driver oncogenes in CRC, we carried out an outlier expression analysis focused on protein kinases [24] , as the latter are frequently implicated in cancer and are ideally suited for therapeutic inhibition. Of the 448 kinase genes expressed in the data set [25] , 32 (7.1%) displayed an outlier expression profile. A striking increase in the prevalence of outliers was observed in the tyrosine kinase (TK) subfamily (15 out of 74, 2.84 × enrichment, hypergeometric P value <0.0001). Of these 15 TKs, nine were outliers only in RAS/BRAF wild-type cells, and were therefore named «WT specific». The enrichment for WT-specific outliers in the TK subgroup was significant (9 out of 15, 3.21 × enrichment, hypergeometric P value<0.0005). Interestingly, eight out of the nine WT-specific outlier TKs clustered in cell lines resistant to cetuximab. The list of WT-specific outliers’ genes comprises ALK , FER , FGFR2 , KIT , NTRK1 , NTRK2 , PDGFRA and RET ( Fig. 4a ). 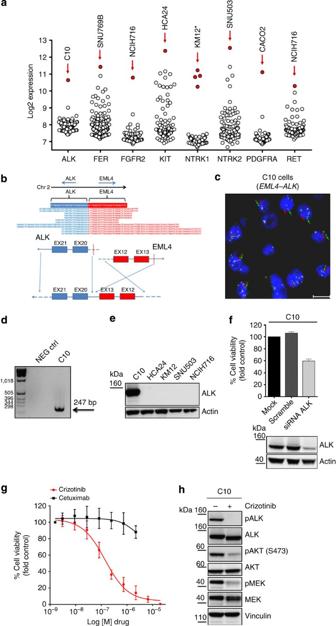Figure 4: Identification of outlier kinase genes in 151 CRC cell lines. (a) Scatter-plot representation of transcriptional outlier kinases in 151 CRC cells. Coloured circles represent outlier kinases with >5 s.d. and >5-fold differential expression compared with median expression. Asterisk labels the KM12 family of cells—KM12, KKM12C, KM12SM and KM12L4. (b) RNA-seq analysis unveiled an in-frame gene fusion event between exon 20 of theALKgene and the exon 13 of theEML4gene on chromosome 2 in the C10 CRC cell line. (c) Break-apart FISH analysis ofALKin C10 cells shows clear separation of green (5′) and red (3′) signals corresponding to theALKgene (original × 63 magnification; scale bar, 10 μm). Scale bars, 10 μm (d) PCR on the cDNA of C10 cells confirmed the EML4–ALK translocation. (e) Western blot analysis confirmed overexpression of ALK protein in C10 cells, at a molecular weight compatible with anEML4–ALKgenetic rearrangement. (f) RNAi knockdown of ALK inhibits cell proliferation of C10 cell line harbouring theEML4–ALKfusion gene. C10 cells were analysed by ATP lite proliferation assay 5 days after transfection with ALK-specific pooled siRNAs, scrambled siRNA or transfection reagent (mock). Data are expressed as average±s.d. of three independent experiments. siRNA-mediated downregulation of ALK levels were verified by western blot analysis. (g) C10 cells, resistant to the EGFR inhibitor cetuximab, are sensitive to the ALK inhibitor crizotinib. Cell viability was assessed by measuring ATP content after 5 days of treatment. Data are expressed as average±s.d. of three independent experiments. (h) Crizotinib treatment downregulates MAPK and PI3K pathways in C10 cells harbouring theALKgenetic rearrangement. C10 cell lines were treated with crizotinib (an ALK inhibitor) for 12 h, after which whole-cell extracts were subjected to western blot analysis. Figure 4: Identification of outlier kinase genes in 151 CRC cell lines. ( a ) Scatter-plot representation of transcriptional outlier kinases in 151 CRC cells. Coloured circles represent outlier kinases with >5 s.d. and >5-fold differential expression compared with median expression. Asterisk labels the KM12 family of cells—KM12, KKM12C, KM12SM and KM12L4. ( b ) RNA-seq analysis unveiled an in-frame gene fusion event between exon 20 of the ALK gene and the exon 13 of the EML4 gene on chromosome 2 in the C10 CRC cell line. ( c ) Break-apart FISH analysis of ALK in C10 cells shows clear separation of green (5′) and red (3′) signals corresponding to the ALK gene (original × 63 magnification; scale bar, 10 μm). Scale bars, 10 μm ( d ) PCR on the cDNA of C10 cells confirmed the EML4–ALK translocation. ( e ) Western blot analysis confirmed overexpression of ALK protein in C10 cells, at a molecular weight compatible with an EML4–ALK genetic rearrangement. ( f ) RNAi knockdown of ALK inhibits cell proliferation of C10 cell line harbouring the EML4–ALK fusion gene. C10 cells were analysed by ATP lite proliferation assay 5 days after transfection with ALK-specific pooled siRNAs, scrambled siRNA or transfection reagent (mock). Data are expressed as average±s.d. of three independent experiments. siRNA-mediated downregulation of ALK levels were verified by western blot analysis. ( g ) C10 cells, resistant to the EGFR inhibitor cetuximab, are sensitive to the ALK inhibitor crizotinib. Cell viability was assessed by measuring ATP content after 5 days of treatment. Data are expressed as average±s.d. of three independent experiments. ( h ) Crizotinib treatment downregulates MAPK and PI3K pathways in C10 cells harbouring the ALK genetic rearrangement. C10 cell lines were treated with crizotinib (an ALK inhibitor) for 12 h, after which whole-cell extracts were subjected to western blot analysis. Full size image Outlier kinase genes are therapeutic targets in CRC cells We next performed genetic and functional validation of the TK outliers. We decided to focus on TKs for which targeted agents are in clinical trial or are already approved for treatment, namely ALK, FGFR2, KIT, NTRK1, NTRK2, RET and PDGFRA. This analysis revealed that the overexpression of NTRK1 and FGFR2 is associated to molecular alterations, such as gene translocation ( NTRK1 ) or gene amplification ( FGFR2 ; Supplementary Figs 5 and 6 ), previously described in cellular models and in cancer patients [26] , [27] , [28] , thus validating the experimental approach. The other TK outlier genes were not previously reported in CRC cells. We detected an in-frame gene fusion event between exon 20 of ALK and exon 13 of EML4 in C10 cells ( Fig. 4b ). Break-apart fluorescent in situ hybridization (FISH), complementary DNA (cDNA) PCR and western blot analysis confirmed the EML4–ALK translocation in C10 cells ( Fig. 4c–e ). We reasoned that if the outlier kinase genes were causally implicated as oncogenic drivers, they should be functionally relevant in the corresponding cell models. We also postulated that the functional dependencies would be cell specific. To formally test these possibilities, we used two complementary approaches—reverse genetics and pharmacological inhibition. Candidate-specific gene suppression was achieved with short interfering RNA (siRNA). In all cases, reduced protein expression of the ‘outlier’ TK resulted in significant impairment of cell growth, which was often accompanied by downstream signalling inhibition and apoptosis ( Fig. 4f ; Supplementary Figs 5–8 ). Pharmacological validation of the TK outliers was performed using the following kinase-targeted drugs—CEP701 (TRK inhibitor), AZD4547 (FGFR2 inhibitor), crizotinib (ALK inhibitor), ponatinib (RET inhibitor) and imatinib and nilotinib (KIT and PDGFRA inhibitor). The drug inhibition profiles were cell specific and paralleled the expression profiles of individual TKs confirmed by RNA-seq in the corresponding cell models ( Figs 4g,h and 5 and Supplementary Figs 5–8 ). In two cases (KIT and PDGFRA) drug inhibition did not affect cell growth ( Supplementary Fig. 8d,h ). Nonetheless, in KIT-overexpressing cells, a reverse genetic experiment revealed functional dependency ( Supplementary Fig. 8b,c ). 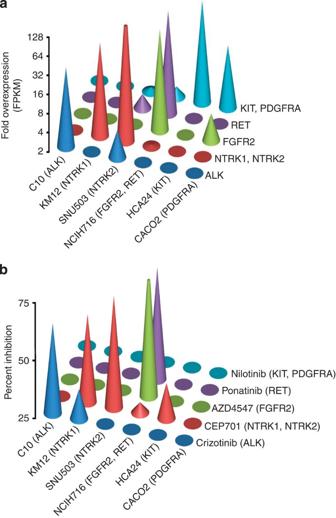Figure 5: Overexpressed kinase genes are therapeutic targets in CRC. (a) RNA-seq analysis of the indicated cell lines shows the overexpression of TK outlier originally identified by microarray data analysis. FPKM, fragments per kilobase of exon per million fragments mapped. (b) Drug profiling with kinase inhibitors. The indicated cell lines were treated with crizotinib (ALK inhibitor) 240 nM, CEP701 (TRK inhibitor) 100 nM, AZD4547 (FGFR inhibitor) 100 nM, ponatinib45(RET inhibitor) 100 nM or nilotinib (KIT and PDGFRA inhibitor) 240 nM for 5 days. Viability was then assessed by measuring ATP content. Figure 5: Overexpressed kinase genes are therapeutic targets in CRC. ( a ) RNA-seq analysis of the indicated cell lines shows the overexpression of TK outlier originally identified by microarray data analysis. FPKM, fragments per kilobase of exon per million fragments mapped. ( b ) Drug profiling with kinase inhibitors. The indicated cell lines were treated with crizotinib (ALK inhibitor) 240 nM, CEP701 (TRK inhibitor) 100 nM, AZD4547 (FGFR inhibitor) 100 nM, ponatinib [45] (RET inhibitor) 100 nM or nilotinib (KIT and PDGFRA inhibitor) 240 nM for 5 days. Viability was then assessed by measuring ATP content. Full size image Translocation of ALK and NTRK1 genes in CRC samples To establish the clinical relevance of the cell line-based findings, we assessed whether the outlier TKs might be identified in CRC specimens using the same methodology. To this end, we downloaded from cBbioPortal [29] , [30] ( http://www.cbioportal.org ) the RNA-seq expression Z scores for 352 CRC tissue samples generated by the Cancer Genome Atlas (TCGA) network [5] . The entire set of candidates described above, with the exception of KIT, was independently validated as RNA expression outliers in the TCGA CRC data set ( Fig. 6a ). As a further validation, we verified whether the ‘outlier’ strategy could lead to retrieval of TK candidates in archival CRC specimens for which RNA is typically not readily available. In this scenario, the most practical screening method should be capable of interrogating protein (rather than RNA) expression, on formalin-fixed paraffin-embedded (FFPE) samples. As a proof of principle, we focused on NTRK1 /Trk-A and ALK. An immunohistochemistry (IHC)-based screen was applied to 742 CRC FFPE samples using a Trk-A (the protein encoded by NTRK1 gene)-specific antibody. One Trk-A outlier sample was unequivocally identified ( Fig. 6b,c ). The IHC profile was followed by break-apart FISH analysis, which detected NTRK1 genetic rearrangement in the TrK-A positive sample ( Fig. 6d ). Screening with and ALK-specific antibody of 742 CRC FFPE retrieved a sample with high levels of the ALK protein ( Fig.6e,f ). In the same specimen, break-apart FISH highlighted a genetic translocation involving the ALK gene ( Fig. 6g ). 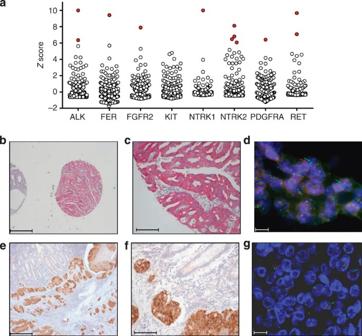Figure 6: NTRK1 and ALK molecular alterations in CRC specimen. (a) Scatter plot representation of transcriptional outlier kinases in 352 CRC tissue samples from the TCGA database. Red circles highlight samples withZ-scoresvalues>6. (b–c) Immunohistochemistry based identification of FFPE CRC displaying Trk-A protein overexpression. 1/742 samples was markedly positive for Trk-A overexpression (d) Break-apart FISH analysis revealedNTRK1gene rearrangement in the FFPE sample positive by IHC. (e–f) Immunohistochemistry based identification of FFPE CRC displaying ALK protein overexpression. 1/742 samples was markedly positive for ALK overexpression. (g) Break-apart FISH analysis revealed ALK gene rearrangement in the FFPE sample positive by IHC. Panelsb,eoriginal 4 × magnification, scale bar=500 μm; panelsc,foriginal 20 × magnification, scale bar=100 μm; panelsd,goriginal 63 × magnification, scale bar=10 μm. Figure 6: NTRK1 and ALK molecular alterations in CRC specimen. ( a ) Scatter plot representation of transcriptional outlier kinases in 352 CRC tissue samples from the TCGA database. Red circles highlight samples with Z-scores values>6. ( b – c ) Immunohistochemistry based identification of FFPE CRC displaying Trk-A protein overexpression. 1/742 samples was markedly positive for Trk-A overexpression ( d ) Break-apart FISH analysis revealed NTRK1 gene rearrangement in the FFPE sample positive by IHC. ( e – f ) Immunohistochemistry based identification of FFPE CRC displaying ALK protein overexpression. 1/742 samples was markedly positive for ALK overexpression. ( g ) Break-apart FISH analysis revealed ALK gene rearrangement in the FFPE sample positive by IHC. Panels b , e original 4 × magnification, scale bar=500 μm; panels c , f original 20 × magnification, scale bar=100 μm; panels d , g original 63 × magnification, scale bar=10 μm. Full size image Human neoplasms are highly heterogeneous, and clinical evidence indicates that pharmacogenetic relationships often involve oncogenic events occurring at low prevalence. Accordingly, precision oncology depends on the ability to functionally interrogate preclinical models capturing the molecular heterogeneity observed in patients. While collections of cancer cells derived from multiple tumor types have been previously described [1] , [2] , [4] , comprehensive databases of cells derived from single tumour lineages are much less common [16] , [31] . To capture the clinical heterogeneity of CRCs, we assembled a collection of 151 cell lines. Notably, genetic finger printing and transcriptional profiling highlighted that several CRC lines previously thought to be unrelated are in fact derived from the same individual. This finding should be helpful in designing future studies and may facilitate the interpretation of previous analysis involving ‘redundant’ cell models. The clinical relevance of the cell database was confirmed by showing that common oncogenic events ( KRAS , NRAS , BRAF , PIK3CA and PTEN alterations) are present in the collection at rates similar to those found in CRC patients. Previous studies evaluated sensitivity to EGFR blockade (with the anti-EGFR antibody cetuximab) in a fraction of the CRC lines described in this work [32] . We found a strong concordance among measurements obtained in independent laboratories, indicating that sensitivity to EGFR inhibition is a stable phenotype of colorectal tumours. While the molecular determinants of EGFR sensitivity are presently unknown, our data suggest a prominent intrinsic (cell autonomous) component. We conclude that genetic and pharmacological profiling CRC lines can successfully nominate clinically-relevant molecular determinants of response to targeted therapies. In addition to the mutation-based categories described above, CRC can be subdivided in up to six transcriptional subtypes with distinct molecular and clinical features [8] , [9] , [10] , [11] , [12] , which we found to be robustly maintained in cells grown in vitro . This observation, along with the evidence that independent cell lines derived from the same patient consistently co-cluster transcriptionally, suggests that the transcriptional profile is stable and predominantly controlled by the genome in the absence of environmental inputs. These results further support the functional correspondence of CRC cell panel described here with CRC specimens. Previous studies have also suggested that transcriptional CRC subtypes may be associated with drug response. The cell models described here recapitulated the association between response to EGFR inhibitors and enrichment for the TA transcriptional class, which was identified in CRC clinical samples [12] . Along this line, the classification of cells we present will facilitate future screenings with chemical or RNA interference libraries aimed at identifying novel pharmacogenomic relationships in specific transcriptional subtypes. We previously reported that a subset of colorectal tumours, in which resistance to EGFR blockade occurs in a RAS/RAF wild-type background, display overexpression of two TK genes, HER2 or MET [33] , [34] . In 41/151 lines, which were analysed in this study, the mechanism of resistance to cetuximab is unaccounted for. We hypothesized that in some of these cells resistance might likewise be driven by the overexpression of a kinase gene. We therefore employed an outlier analysis based on expression levels of TK genes to identify additional kinase (and therefore actionable) targets in the subset of WT RAS/BRAF CRC cells intrinsically resistant to EGFR therapies. Seven of the TKs retrieved by this approach (ALK, FGFR2, KIT, NTRK1, NTRK2, RET and PDGFRA) are the target of drugs undergoing clinical testing or approved. In some instances (FGFR2, ALK or NTRK1), overexpression of the TK gene was associated with amplification or translocation of the corresponding locus. The same genetic alterations have been previously reported in CRC cells and patients [26] , [27] , [28] , thus validating our approach. Our data further suggest that overexpression of TK sustains primary resistance to EGFR blockade, and could be used to identify patients unlikely to respond to cetuximab or panitumumab. Of note, with the exception of RET and FGFR2, which coexisted in NCIH716 cells, outlier expression of TKs was mutually exclusive. Our results have broad implications for the use of kinase inhibitors in CRCs and potentially other cancer types. First, companion diagnostic assays are essential to identify those (rare) patients with tumours bearing aberrantly expressed kinases. Since the molecular events leading to protein overexpression can be multiple (gene amplification, gene fusions and translocations with different partners and break points), we propose that IHC should be better suited than other methods to serve this purpose. As a test case, we demonstrated the feasibility of this approach to identify CRC patients carrying overexpressed and genetically altered Trk-A and ALK kinases. Additional work is warranted to develop and validate IHC assays for the other outlier TK genes. Importantly, given the low prevalence of these outlier events, strategies aimed at concomitantly screen for multiple molecular alterations should be implemented. Eventually, it is likely that next-generation sequencing will become the most effective approach to detect molecularly deregulated kinase genes as it allows concomitant assessment of single-nucleotide variants as well as a gene copy number alterations and translocations. Our results also highlight the relevance of clinical trials involving CRC patients carrying molecularly altered TK genes, which can be readily identified using FFPE specimens. Our data suggest that these patients are unlikely to benefit from anti-EGFR antibodies but likely to profit from currently available drugs such as ALK and TRK inhibitors. It is important to note that in some instances (that is, KIT), blockade of the kinase activity with a specific kinase inhibitor did not impair growth, while TK suppression with siRNA revealed functional dependency and triggered apoptosis. This suggests that downregulation of the candidate protein, for example, through specific antibodies, might be necessary in some instances. Our data further suggest that TK inhibitors effectively impair tumour growth in cell lines in which transcriptional deregulation is accompanied by the genetic activation of the kinase (TRK, ALK and FGFR2), but not in the cell lines where no genetic activation was identified (PDGFR and KIT). In conclusion, our results describe a powerful preclinical resource capturing the heterogeneity of CRC patients, which can be used to define multidimensional information of clinical relevance and applicability. Cell lines and reagents A collection of 152 cell lines of intestinal origin was assembled from different worldwide cell line banks or academic laboratories as indicated in Supplementary Data 1 . All cell lines were maintained in their original culturing conditions according with supplier guidelines. Cells were ordinarily supplemented with fetal bovine serum at different concentrations, 2 mM L -glutamine, antibiotics (100 U ml −1 penicillin and 100 mg ml −1 streptomycin) and grown in a 37 °C and 5% CO 2 air incubator. Cells were routinely screened for absence of Mycoplasma contamination using the Venor GeM Classic kit (Minerva Biolabs). The identity of each cell line was checked by Cell ID System and by Gene Print 10 System (Promega), throught STR at 10 different loci (D5S818, D13S317, D7S820, D16S539, D21S11, vWA, TH01, TPOX, CSF1PO and amelogenin). Amplicons from multiplex PCRs were separated by capillary electrophoresis (3730 DNA Analyzer, Applied Biosystems) and analysed using GeneMapperID software from Life Technologies. Resulting cell line STR profiles were cross-compared and matched with the available STR from ATCC, DSMZ, JCRB, Korean Cell Line Bank, ECCAC and CellBank Australia repositories online databases. Results of the analysed loci for each cell line are provided in Supplementary Data 1 . Cetuximab was obtained from the Pharmacy at Niguarda Ca’ Granda Hospital in Milan, Italy; Crizotinib, AZ4547, imatinib, ponatinib and nilotinib were purchased from Selleck Chemicals. CEP701 was purchased from Sigma-Aldrich. DNA analysis Genomic DNA samples were extracted by Wizard SV Genomic DNA Purification System (Promega). The MSI status has been evaluated by mean of MSI Analysis System kit (Promega). The analysis requires a multiplex amplification of seven markers including five mononucleotide repeat markers (BAT-25, BAT-26, NR-21, NR-24 and MONO-27) and two pentanucleotide repeat markers (Penta C and Penta D). The products were analysed by capillary electrophoresis in a single injection (3730 DNA Analyzer, ABI capillary electrophoresis system (Applied Biosystems). The results were analysed using GeneMarker V2.2.0 software. As cell lines do not have a corresponding normal tissue available for comparison, their profile has been analysed with an MSS cell line of control, K562. Samples with instability in one, two or more markers (mononucleotide repeat) are defined as MS-instable (MSI). Samples with no detectable alterations are MS-stable (MSS). The same samples of genomic DNAs were used for PCR amplification to check 16 hotspot CRC mutations in all cells (reported in Supplementary Data 1 ). The mutational status of KRAS (exons 2, 3 and 4), NRAS (exons 2 and 3), HRAS (exons 2 and 3), BRAF (exon 15) and PIK3CA (exons 9 and 20) was determined by Sanger sequencing (primers’ sequences are listed in Supplementary Data 3 ). RNA extraction and gene expression profiling RNA was extracted using miRNeasy Mini Kit (Qiagen), according to the manufacturer’s protocol. The quantification and quality analysis of RNA was performed on a Bioanalyzer 2100 (Agilent), using RNA 6000 nano Kit (Agilent). Synthesis of cDNA and biotinylated cRNA was performed using the IlluminaTotalPrep RNA Amplification Kit (Ambion), according to the manufacturer’s protocol using 500 ng of total RNA. Quality assessment and quantification of cRNAs were performed with Agilent RNA kits on Bioanalyzer 2100. Hybridization of cRNAs (750 ng) was carried out using Illumina Human 48 k gene chips (Human HT-12 V4 BeadChip). Array washing was performed using Illumina High Temp Wash Buffer for 10′ at 55 °C, followed by staining using streptavidin-Cy3 dyes (Amersham Biosciences). Probe intensity data were obtained using the Illumina Genome Studio software (Genome Studio V2011.1). Raw data were Loess normalized with the Lumi R package and further processed with Excel software. Tissue of origin analysis Thirty panels of genes with tissue-specific expression were retrieved from the TIGER portal [13] ( http://bioinfo.wilmer.jhu.edu/tiger/ ) and filtered to remove gene symbol redundancies. Similarly, to avoid probe redundancy in array data, when multiple probes matched the same gene we selected the one with the highest s.d.. For the tissue of origin analysis, we assumed that the vast majority of the cell lines present in this data set were of colorectal origin, while only a very small fraction could possibly derive from other tissues. Therefore, to increase sensitivity of the colon-specific gene panel, genes not expressed (L2S<9) in at least 50 of the 152 CRC cells were removed from the panel. To increase the specificity of other tissue-specific gene panels, genes from these panels expressed (L2S>9) in more than three CRC cell lines (2%) were also removed. For each gene of a tissue-specific panel, the TIGER database provided an ‘EST Enrichment’ (EE) score, proportional to the extent of tissue specificity. To give more weight to genes with high EE score in the estimation of the tissue of origin, EE scores were squared and summed. Then, the squared EE score of each gene was divided by the sum, to obtain a ‘Scaled EE score’ representing what fraction of the tissue specificity of the gene panel is brought by each individual gene. Finally, a ‘tissue score’ was calculated for each gene panel by summing the products of gene expression and scaled EE score, and using the resulting value as exponential of 2 to obtain linear values. Unsupervised expression clustering After removing the COLO741 melanoma cell line from the data set, we assessed global transcriptional correlations across the remaining 151 cell lines by unsupervised clustering A detection filter was applied to the 151 cell line data set by requesting that the reported detection P value reported in GSE59857 was zero in at least one of the 151 samples. After detection filtering, when multiple probes matched the same gene, we selected the one with the highest s.d. This led to the identification of 19,828 unique genes detected in at least one cell line. Before clustering, we applied a further filter based on s.d. across samples (s.d. of Log 2 Signal>0.8). We then employed the Log 2 signal of 3,132 genes passing this filter for hierarchical clustering with maximum linkage based on Pearson correlation, using the GEDAS software [35] . Drug proliferation assay CRC cell lines were seeded at different densities (2–4 × 10 3 cells per well) in 100 μl complete growth medium in 96-well plastic culture plates at day 0. The following day, serial dilutions of the indicated drugs were added to the cells in serum-free medium, while medium-only (in case of cetuximab) or dimethylsulphoxide-only (for all the other drugs)-treated cells were included as controls. Plates were incubated at 37 °C in 5% CO 2 for 4 or 5 days, after which the cell viability was assessed by measuring ATP content through Cell Titer-Glo Luminescent Cell Viability assay (Promega). Luminescence was measured by Perkin Elmer Victor X4. On the basis of cell viability after 4 days of treatment with clinical relevant concentration of 10 μg ml −1 of cetuximab and on the shape of the drug screening-cell response growth curves, CRC cells were defined sensitive when cell viability was ≤40% at 10 μg ml −1 of cetuximab. We then calculated the AUC for each cell line of the panel and selected the threshold of AUC index ≥13,000 based on the values of AUC obtained in the subgroup of sensitive cell lines. The area under the concentration–inhibition curve (index AUC) was computed using Excel [36] . The ‘cetuximab effect arbitrary index’ was calculated by subtracting the threshold value of 13,000 from the AUC index of each cell line to highlight the subpopulation of sensitive cell lines (those with a negative index). Classification of CRC cell lines into intrinsic subtypes To classify cell lines into CRC subtypes according to previously published transcriptional classification systems, gene lists for the five classifiers were obtained from the supplementary information of the relevant publications. We then employed the NTP algorithm [23] on the 151 CRC lines expression data set of 19,828 genes described above. NTP is a nearest neighbour classifier developed to classify samples with defined gene signatures also when generated in a different microarray platform, and to provide an estimate of classification robustness by computing FDR and P value. NTP analysis was conducted using the GenePattern Bioportal [37] ( http://www.broadinstitute.org/cancer/software/genepattern/ ). For NTP implementation, we selected genes positively and specifically associated to one subtype. The CRC subtype classifiers were generated by different procedures. To perform reciprocal comparisons in an independent data set, based on a different microarray platform, we had to adapt them to a common classification strategy. The thresholds for gene selection described below were chosen to remove genes with low class discrimination power (to improve sensitivity and specificity), while at the same time maintaining a reasonable number of classifying genes (for the stability and platform independence of the classifier). De Sousa [9] and Sadanandam [12] gene signatures have originally been defined using the same approach, that is, significance analysis of microarrays [38] followed by prediction analysis for microarrays (PAM) [39] , to build lists of genes positively or negatively associated to each molecular subtype. The extent and sign of association is represented by the PAM score. To select only genes with a strong positive association to one class, we associated each gene to the class corresponding to the maximum PAM value, and only if the difference between the maximum and second highest value was sufficiently high (>0.1). Subtype signatures of the Marisa [10] classifier were defined by filtering the list of 1,108 genes provided in Supplementary Table S10 of their work, using the associated log fold changes and adjusted P values for each gene in each of the six CRC subtypes. In particular, we assigned a gene to a class signature if two conditions were met: (i) its fold change in the class was the highest among its fold changes in all the classes; (ii) the adjusted P value in the same class was the minimum between the adjusted P values of all the other classes with a positive fold change. As done for De Sousa and Sadanandam classifiers, to select only genes with a strong association to a single subtype, we selected only those genes having a difference between the highest and second highest log fold change greater than 0.2. The Roepman [11] signatures were defined based on positive genes provided in Table 2 of the original work. The Budinska [8] gene signatures were provided on Table 1 of the original work as metagenes, each with statistical assessment of differential expression across subtypes. Adaptation to NTP required two steps: (i) selection of the metagenes specifically upregulated in each subtype and (ii) extraction of the lists of genes belonging to the selected metagenes. A metagene was associated with a subtype if it was significantly upregulated in that subtype, had the highest positive fold change (Log2 ratio versus median) in that subtype and if the difference against the second highest subtype was greater than a log2 ratio of 0.2. Then, for each subtype, the lists of genes belonging to the specifically upregulated metagenes were merged to build the subtype signatures. To compare the results obtained by the five different classifiers employed, we computed hypergeometric tests performing a paired-sample enrichment analysis, with Bonferroni correction of the resulting P values. Associations between CRC subtypes and MSI status, BRAF/KRAS mutations and cetuximab sensitivity were evaluated by hypergeometric distribution analysis and Fisher’s exact test. Outlier expression analysis Outlier analysis was performed starting from the 151 CRC lines expression data set. Expression of a gene in a cell line was considered outlier if it was both >5 s.d. and >5-fold greater than its median expression across all cells. Kinase-encoding genes were obtained from ( http://kinase.com/human/kinome/ ) [25] , after annotation with updated gene symbols and mapped on the detection-filtered expression data set of 19,828 unique genes described above. Gene copy number analysis CRC cell lines were trypsinized, washed with PBS and centrifuged; pellets were lysed and DNA was extracted as described above. Real-time PCR was performed with 10 ng of DNA per single reaction using GoTaq QPCR Master Mix (Promega) with an ABI PRISM 7900HT apparatus (Applied Biosytems; primers’ sequences are available on request). Gene copy numbers were normalized to a control diploid cell line, HCEC [40] . siRNA screening The siRNA targeting reagents were purchased from Dharmacon, as a SMARTpool of four distinct siRNA species targeting different sequences of the target transcript. Cell lines were grown and transfected with SMARTpool siRNAs using RNAiMAX (Invitrogen) transfection reagents following the manufacturer’s instructions. In brief, RNAi screening conditions were as follows—on day one, siRNAs were distributed in each well of a 96-wellplate at final concentration of 20 nmol l −1 . Transfection reagents were diluted in OptiMEM and aliquoted at 10 μl per well; after 20 min of incubation, 70 μl of cells in media without antibiotics were added to each well. After 5 days, cell viability was estimated with a luminescent assay measuring cellular ATP levels with CellTiter-Glo Luminescent Assay (Promega). Each plate included the following controls: mock control (transfection lipid only), AllStars (Qiagen) as negative control; Polo-like Kinase 1 (Dharmacon) as positive control [41] . siRNA sequences are listed in Supplementary Data 4 . RNA-seq Total RNA extracted from C10, KM12, SNU503, HCA24, CACO2 and NCIH716 cells was processed for RNA-seq analysis with Ion TotRNA Seq kit v2 following the manufacturer’s instruction and sequenced with the Ion Proton System (Ambion—Life Technology). Each fastq file was realigned using Tophat2 v2.0.11 (ref. 42 ). Version hg19 of the genome was used and Gencode v19 as reference transcriptome database. The average value of the reads aligned by Tophat2 is 61%. The fragments per kilobase of exon per million fragments mapped was computed on the aligned reads using Cufflinks software v2.2.1 (ref. 43 ). Moreover, each fastq file was analysed by FusionMap software v 7.0.1.25 (ref. 44 ) obtaining the list of fusion transcripts for each cell line. Immunohistochemistry FFPE CRC samples were available through the clinical database of Ospedale Niguarda and Istituto Nazionale Tumori Regina Elena. Additional CRC specimens’ tissue microarrays were purchased from Abcam (Cat. ab128127). Trk-A and ALK protein expression was evaluated by IHC performed on 3–4 μm-thick tissue sections, using specific antibodies to assess Trk-A expression, the monoclonal antibody (Clone ID EP1058Y, Epitomics, dilution 1:200), which recognizes the carboxyl-terminal portion of the protein was used and the analysis was performed with the automated system BenchMark Ultra (Ventana Medical System Inc., Roche) according to the manufacturer’s instructions, with minimum modifications. Samples were incubated with the primary antibody for 1 h at 42 °C, after which a chromogenic reaction was performed using the ultraView Universal Alkaline Phosphatase Red Detection kit (Ventana, Roche). ALK protein expression was detected using the anti-ALK mouse monoclonal antibody (clone 5A4), which recognizes the intracellular region of ALK. The analysis was performed manually, using N- Histofine ALK Detection Kit, according to the manufacturer’s instructions (Nichirei Biosciences Inc.). Samples were incubated with the primary antibody for 30 min at room temperature and DAB was used as chromogen. For both proteins, specimens were considered positive when the expression was strong and cytoplasmic and present in at least 10% of cells. Healthy tissue, that is, normal colon mucosa, was used as internal negative control. Images were captured with the AxiovisionLe software (Zeiss) using an Axio Zeiss Imager 2 microscope (Zeiss). FISH analysis Tissue sections and cyto-embedded cell lines for fluorescent in situ hybridization (FISH) experiment were prepared according to the manufacturer’s instructions of Histology FISH Accessory kit (Dako). For both types of samples (tissue and cell lines), the last steps before hybridization were: dehydration in ethanol series (70, 90 and 100%), three washes (5′ each) and air drying. To identify the possible NTRK1 gene rearrangements, a dual-colour break-apart probe has been designed a contiguous of two BAC (bacterial artificial chromosome; http://genome.ucsc .) probes, RP11-349I17(1q23.1) and RP11-1038N13 (1q23.1), all together spanning an ∼ 335 kb region encompassing the NTRK1 gene. A dual-colour FISH analysis was performed using respectively: 10 μl mix-probe made up by 1.5 μl BAC genomic probe RP11-349I17 (1q23.1) labelled in Spectrum Orange (Empire Genomics), 1.5 μl BAC genomic probe RP11-1038N13 (1q23.1) labelled in SpectrumGreen and 7 μl LSI-WCP hybridisation buffer (Vysis) for each slide. To identify possible ALK gene rearrangements, an LSI ALK (2p23) Dual-Colour, Break-Apart (Vysis) probe was used. Probes and target DNA of specimens were co-denatured in HYBRite System (DakoGlostrup) respectively at 75 °C for 5 min using NTRK1 probe and at 73° for 5 min for ALK probe, therefore hybridized overnight at 37 °C. Slides were washed with post-hybridization buffer (DakoGlostrup) at 73 °C for 5 min and counterstained wit 4′,6-diamino-2phenylindole (Vysis, Downers Grove, IL. USA). FISH signals were evaluated with a Zeiss Axioscope Imager. Z1 (Zeiss) equipped with single and triple band-pass filters. Images for documentation were captured with CCD camera and processed using the MetaSystems Isis software. Samples were scored as positive either for NTRK1 or ALK gene’s rearrangement when a split signal of the probes was observed, in at least 15% of 100 cells analysed in 10 different fields. Healthy tissue, that is, normal colon mucosa, was used as internal negative control. Western blotting analysis Before biochemical analysis, all cells were grown in their specific media supplemented with 10% fetal bovine serum. Total cellular proteins were extracted by solubilizing the cells in EB buffer (50 mM Hepes pH 7.4, 150 mM NaCl, 1% Triton-X-100, 10% glycerol, 5 mM EDTA, 2 mM EGTA; all reagents were from Sigma-Aldrich, except for Triton-X-100 from Fluka) in the presence of 1 mM sodium orthovanadate, 100 mM sodium fluoride and a mixture of protease inhibitors. Extracts were clarified by centrifugation, normalized with the BCA Protein Assay Reagent kit (Thermo). Western blot detection was performed with enhanced chemiluminescence system (GE Healthcare) and peroxidase conjugated secondary antibodies (Amersham). The following primary antibodies were used for western blotting (all from Cell Signaling Technology, except where indicated): anti-FGFR2 (1:1000); anti-ALK; anti-Trk-A (Santa Cruz; 1:500); anti-Trk (Santa Cruz; 1:500); anti-cKIT (1:1,000); anti-PDGFRA (1:1,000); anti-phospho-p44/42 ERK (Thr202/Tyr204; 1:1,000); anti-p44/42 ERK (1:1,000); anti-phospho-MEK1/2 (Ser217/221; 1:1,000); anti-MEK1/2 (1:1,000); anti-phospho AKT (Ser473; 1:1,000); anti-AKT (1:1,000); anti-PARP (1:1,000); anti-actin (Santa Cruz; 1:3,000); anti-vinculin (Millipore; 1:5,000); anti-PTEN (1:1,000). Anti-RET antibody [45] (1:500) was kindly provided by Professor Massimo Santoro (Federico II, Naples). The full-length western blot membranes are shown in Supplementary Figs 9–13 . Accession codes: Gene expression microarray data have been deposited in the GEO database with accession number GSE59857 How to cite this article: Medico, E. et al. The molecular landscape of colorectal cancer cell lines unveils clinically actionable kinase targets. Nat. Commun. 6:7002 doi: 10.1038/ncomms8002 (2015).